Chemical reactivation of quenched fluorescent protein molecules enables resin-embedded fluorescence microimaging Resin embedding is a well-established technique to prepare biological specimens for microscopic imaging. However, it is not compatible with modern green-fluorescent protein (GFP) fluorescent-labelling technique because it significantly quenches the fluorescence of GFP and its variants. Previous empirical optimization efforts are good for thin tissue but not successful on macroscopic tissue blocks as the quenching mechanism remains uncertain. Here we show most of the quenched GFP molecules are structurally preserved and not denatured after routine embedding in resin, and can be chemically reactivated to a fluorescent state by alkaline buffer during imaging. We observe up to 98% preservation in yellow-fluorescent protein case, and improve the fluorescence intensity 11.8-fold compared with unprocessed samples. We demonstrate fluorescence microimaging of resin-embedded EGFP/EYFP-labelled tissue block without noticeable loss of labelled structures. This work provides a turning point for the imaging of fluorescent protein-labelled specimens after resin embedding. Resin embedding is a well-developed method and is broadly used as a basic tool for both electron microscopy and light microscopy [1] . It was first used to produce ultrathin sections for transmission electron microscopy in 1949 (ref. 2 ). Resin-embedded tissue has good sectioning properties that help researchers overcome the scattering barrier limits that hinder microscopy for thick tissues [3] , [4] . In recent decades, the green-fluorescent protein (GFP) labelling technique has brought revolutionary breakthroughs to fluorescence imaging. Using this powerful molecular biology technique, GFP can be attached to gene products of interest to visibly label their expression, which enables the analysis of biological function and localization [5] . Unfortunately, the dehydration and exposure to organic solvents involved in the embedding procedure cause quenching of Aequorea victoria GFP and its variants (such as the widely used EGFP and EYFP) [6] , resulting in poor fluorescence signals that can make detection impossible. This makes it difficult to combine the advantages of resin-embedding methods with those of modern molecular labelling techniques. For many years, researchers have attempted to improve the preservation of fluorescence in the resin-embedding procedure by empirically optimizing the embedding protocol [7] , [8] , [9] , [10] , [11] , [12] , [13] . Although quenching still exists, fluorescence signals have been successfully detected and analysed in resin-embedded cultured cells and small tissues for correlative microscopy studies [7] , [8] , [9] , [10] . However, these methods are difficult to transplant to process thick tissue blocks. Efforts on embedding macroscopic tissues have been developed [11] , [12] , [13] ; however, serious fluorescence quenching still exists. Furthermore, the mechanism of fluorescence quenching in the resin-embedding procedure remains unknown. In addition, it is uncertain whether labelled structures can be successfully retained. To address this problem, an essential question needs to be answered: what happens to the fluorescent protein molecules when they are being embedded in resins, which causes significant fluorescence quenching? Can fluorescence quenching be effectively avoided or, if that is not possible, can the fluorescence be recovered? The properties of GFP have been systematically studied in aqueous solutions by previous research groups [6] . The behaviours of GFP in acid, base and denaturant solutions have been investigated [14] , [15] , [16] , [17] , [18] , [19] , [20] , [21] , [22] . We are inspired to trace the behaviours of GFP during the resin-embedding process. We found that, instead of direct denaturation, GFP molecules experienced a transition into a nonfluorescent state because of chromophore protonation during resin embedding. Without modifying the normal embedding protocols of the commonly used acryl resins, we find that most of the quenched GFPs can be chemically reactivated to its fluorescent state by post-polymerization processing. We call this process chemical reactivation (CR). The CR method enables reliable preservation of EYFP- and EGFP-labelled structures in resin-embedded tissues. Chemical reactivation When treated by alkaline buffer, significant fluorescence recovery was observed on the block-face of a thy1-YFPH mouse brain that was routinely embedded in LR White resin ( Fig. 1a–c ). The diamond-knife-machined block was suffused with alkaline buffer solutions (such as 0.1 M Na 2 CO 3 , pH=11.6), and the fluorescence intensity of the specimen surface was immediately and dramatically enhanced ( Fig. 1a,b ). Quantitative analysis on five independent resin blocks shows an 11.8±0.7-fold enhancement of fluorescence intensity ( Fig. 1c shows a typical one, Supplementary Fig. 1a–d shows other four independent measurements). Additional experiments found that EYFP fluorescence can also be recovered well in other acrylic resins, such as the commonly used glycol methacrylate (GMA) and methyl methacrylate (MMA) ( Supplementary Fig. 2 ). For the MMA- and GMA-embedded thy1-YFPH mouse brain samples that we tested, ~7.5±0.5- and 7.6±0.6-fold fluorescence intensity enhancements were found, respectively ( N =5; Supplementary Fig. 1e–l , Supplementary Fig. 2c,f ). The fluorescence spectra detected before and after fluorescence recovery matched the spectra of the fluorescent proteins in fresh tissue ( Supplementary Fig. 3 ). These results indicate that a large proportion of the chromophores in resin-embedded tissue are transferred into a nonfluorescent state because of unsuitable chemical conditions, rather than directly damaged, since the Na 2 CO 3 buffer we used to penetrate the resin block is too inert to induce redox reactions with the damaged chromophores. 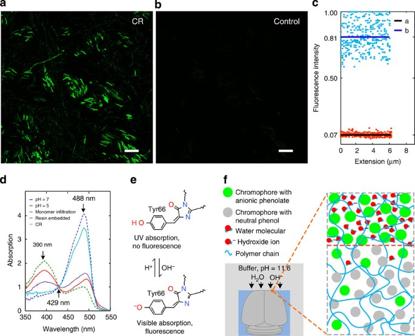Figure 1: Chemical reactivation. Axons in the striatum region of an LR White-embedded P21 thy1-YFPH mouse brain were subjected to chemical reactivation. Different portions of the axons are presented: (a) the chemically reactivated portion; (b) the unaffected portion below the 6-μm chemically reactivated layer. All images are maximum intensity projections of 6-μm-thick z-stacks. (c) The uniform fluorescence intensities of 10 traced axons. This example shows an 11.6-fold enhancement of fluorescence intensity and 11.8±0.7-fold for independent samples (N=5). The blue points show the fluorescence intensity of the chemically reactivated portions of axons along their extensions, and the red points show fluorescence for the unaffected portion. The solid lines (blue or dark) represent the least-squares fitting results for fluorescent intensities. (d) Absorption spectra of EGFP in distilled water (blue, dash line), HAC solution (pH=5, green, dash line), GMA resin monomer (purple), GMA resin polymer (red) and 0.001 M NaOH-penetrated GMA polymer (light blue). (e) Chromophore dynamics during resin embedding and chemical reactivation. (f) The mechanism of the CR phenomenon. Enlargement reveals that water molecules and hydroxide ions penetrate throughout the polymer chain interspaces and act on the EYFP molecules. Scale bar: (a,b) 20 μm. Figure 1: Chemical reactivation. Axons in the striatum region of an LR White-embedded P21 thy1-YFPH mouse brain were subjected to chemical reactivation. Different portions of the axons are presented: ( a ) the chemically reactivated portion; ( b ) the unaffected portion below the 6-μm chemically reactivated layer. All images are maximum intensity projections of 6-μm-thick z-stacks. ( c ) The uniform fluorescence intensities of 10 traced axons. This example shows an 11.6-fold enhancement of fluorescence intensity and 11.8±0.7-fold for independent samples ( N =5). The blue points show the fluorescence intensity of the chemically reactivated portions of axons along their extensions, and the red points show fluorescence for the unaffected portion. The solid lines (blue or dark) represent the least-squares fitting results for fluorescent intensities. ( d ) Absorption spectra of EGFP in distilled water (blue, dash line), HAC solution (pH=5, green, dash line), GMA resin monomer (purple), GMA resin polymer (red) and 0.001 M NaOH-penetrated GMA polymer (light blue). ( e ) Chromophore dynamics during resin embedding and chemical reactivation. ( f ) The mechanism of the CR phenomenon. Enlargement reveals that water molecules and hydroxide ions penetrate throughout the polymer chain interspaces and act on the EYFP molecules. Scale bar: ( a , b ) 20 μm. Full size image Mechanism of EGFP quenching in acryl resin To determine whether a large proportion of chromophores was restored from a nonfluorescent state, we measured the absorption spectra of EGFP after resin monomer infiltration, polymerization and fluorescence recovery. To ensure broad generality of the results, we simply used purified recombinant EGFP (histidine-tagged, expressed in Escherichia coli ). During the embedding processing, only the absorption spectrum of intact EGFP, with peaks at ~390 and 488 nm [21] , [22] , was detected. No shoulders of absorption were observed around 384 and 448 nm, which would indicate denatured or digested GFP [14] , [15] , [16] , [18] , [19] , [20] (purple and red curves in Fig. 1d ). These clean absorption spectra indicate that EGFP denaturation during GMA embedding can be neglected. As the resin monomer infiltrates and polymerizes, the 390-nm absorption peak gradually increases, and the 488-nm peak decreases (purple and red curves in Fig. 1d ). These absorption spectrum changes indicate that a large proportion of the EGFP chromophores change to a nonfluorescent neutral phenol state [17] , [22] , [23] , [24] . When fluorescence was recovered by using alkaline buffer (0.001 M NaOH, pH=11), the absorption spectrum recovered to that of EGFP in neutral buffer, with only one 488-nm absorption peak detected (light blue curve in Fig. 1d ). This dramatic change shows that chromophores transferred into the nonfluorescent neutral phenol state during the embedding procedure can be chemically reactivated to their fluorescent anionic phenolate state. The absorption spectra of EGFP in two other resins (MMA and LR White) were also investigated ( Supplementary Fig. 4 ), and similar absorption spectrum changes were observed. Thus, the mechanism of fluorescence recovery has been identified: the alkaline buffer penetrates into the resin-embedded tissue and ionizes the chromophore phenols that became protonated during the resin-embedding procedure, which reactivates the corresponding quenched EGFP molecules ( Fig. 1e,f ). We refer to this fluorescence recovery as CR. We note that the success of CR theoretically does not depend on the expression host. Our tests show that CR can be successfully induced in other tissues, and even in other species. For example, CR provided an ~8.3-fold fluorescence enhancement in MMA-embedded fruit flies ( Fig. 2 ), enabling imaging of EGFP-labelled fine axon fibres that could not be easily distinguished from background in the normal embedded state. 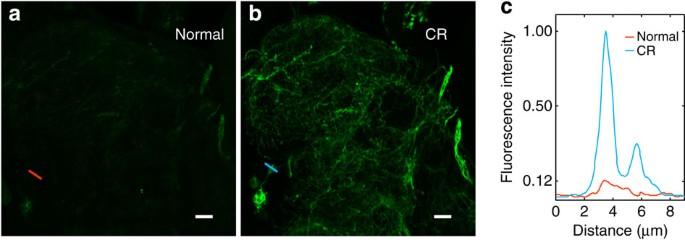Figure 2: CR in a section from an MMA-embedded EGFP-labelled fruit fly. An image of neural fibres in normal MMA-embedded fruit fly is shown before (a) and after (b) CR. There is an ~8.3-fold fluorescence enhancement for labelled structures. (c) Fluorescence intensity plots for the red and blue lines labelled in (a,b). Scale bar: 10 μm. Figure 2: CR in a section from an MMA-embedded EGFP-labelled fruit fly. An image of neural fibres in normal MMA-embedded fruit fly is shown before ( a ) and after ( b ) CR. There is an ~8.3-fold fluorescence enhancement for labelled structures. ( c ) Fluorescence intensity plots for the red and blue lines labelled in ( a , b ). Scale bar: 10 μm. Full size image To confirm that chromophore protonation is the main cause of fluorescence quenching during resin embedding, we measured the EYFP molecular preservation ratio by quantitatively comparing EYFP-labelled structures between the CR-enhanced resin-embedded state and the control state. The control state represents the original paraformaldehyde (PFA)-fixed state immediately before embedding. Here we present the EYFP preservation results for an MMA-embedded section from brain tissue samples ( Fig. 3 ). We have measured a value of 6.84 for the pKa of EYFP in the PFA-fixed thy1-YFPH mouse brain ( Supplementary Fig. 5 ). In the original PFA-fixed tissue (stored in 0.01 M phosphate-buffered saline (PBS), pH=7.4), ~78% of the chromophores were ionized and fluorescent [21] , [25] , [26] . Therefore, we represent the total amount of EYFP molecules in the fixed state structure as 1.28-fold (1/0.78) fluorescence intensity (1.28 I 0 ), and the amount of preserved EYFP molecules as the fluorescence intensity detected after CR procedure ( I ). The EYFP preservation ratio is then represented as I /(1.28 I 0 ) (see Fig. 3e,f,h ). To control for fluorescence intensity enhancement caused by embedding-induced shrinkage, we chose to measure a fine structure in the neuron process, the mushroom spine [27] , which has a large head but narrow neck and stands apart from the dendrite. The fluorescence intensities were integrated over the whole spine body to count all expressed EYFP molecules ( Fig. 3e,f ). To reduce scattering interference to a negligible level, we included only the mushroom spines within the surface layer (a 4-μm-thick layer). On the basis of statistics from 30 mushroom spines, we found that the EYFP preservation ratio in MMA-embedded tissue reached 98% along the extension of a whole layer V pyramidal neuron, and we found that the preservation ratio does not vary greatly according to position ( Fig. 3h ). Regions both near to and far from the edge of the tissue were evaluated separately. The EYFP preservation ratios were 98% at the centre of the tissue (soma-clustering region) and 97% at the edge (apical dendrite region). This difference is negligible compared with the s.d.’s of those measurements (~0.09). As expected, although a large proportion of the EYFP molecules are quenched in the resin-embedding procedure, the chromophore damage is not significant. The same measurements were repeated on GMA- and LR White-embedded thy1-YFPH mouse brain tissues and on GMA-, MMA- and LR White-embedded thy1-GFPM mouse brain tissues. The FP preservation ratios were 97% and 93% for EYFP, and 96%, 88% and 76%, respectively, for EGFP ( Supplementary Fig. 6 ). These high preservation ratios obtained with CR indicate that chromophore protonation is the main cause of fluorescence quenching in the resin-embedding procedure. Our CR method can efficiently switch those protonated chromophores back to their fluorescent anionic state. 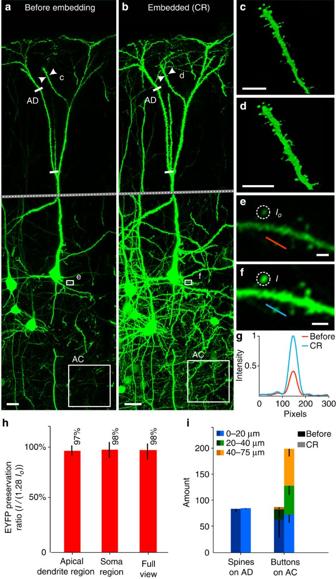Figure 3: Preservation of structure and EYFP fluorescence in CR-enhanced resin-embedded tissue. Image of layer V pyramidal neurons in thy1-YFPH mouse cortex before and after MMA embedding. (a) Paraformaldehyde-fixed state; (b) CR-enhanced embedded state. During imaging, paraformaldehyde-fixed brain slices were kept in phosphate-buffered saline (0.01 M, pH=7.4); the corresponding LR White-embedded brain slices were kept in Na2CO3solution (0.1 M, pH=11.6). All images were acquired on the same microscope (Nikon A1) with the same configuration at 25°C (room temperature). Image dimensions ofbwere enlarged 1.34-fold to correct for the shrinkage caused by the embedding procedure. Intermediate dendrites are abbreviated (grey bands with dashed lines) to allow a much closer view of the details. Images of one apical dendrite were recorded before (c) and after (d) embedding to allow direct comparison of dendritic spine morphology. (e,f) Enlargements of insets (white boxes) froma,b.I0andIrepresent the integration of fluorescence intensities in the corresponding white circle. Fluorescence intensities of pixels crossed by the red and blue lines are plotted (g) as curves of the corresponding colour. (h) The EYFP preservation ratio. At least 15 mushroom spines were measured for every subregion. Error bars represent s.d.’s. (i) Statistics of dendritic spines and collateral boutons before and after embedding. Spines were counted on a portion of apical dendrites (ADs); boutons were counted in a 100 × 100 × 75 μm3layer (measured in the fixed state) containing axon collaterals (AC)s concentrated at three depth intervals (0–20, 20–40 and 40–75 μm). Deep-coloured pillars represent the PFA-fixed state, and light-coloured pillars represent the CR-enhanced resin-embedded state. Error bars represent the number of boutons with uncertain identification. All images are shown with the same colour bar except forc,d. Scale bar: (a,b) 40 μm; (c,d) 10 μm; (e,f) 2 μm. Figure 3: Preservation of structure and EYFP fluorescence in CR-enhanced resin-embedded tissue. Image of layer V pyramidal neurons in thy1-YFPH mouse cortex before and after MMA embedding. ( a ) Paraformaldehyde-fixed state; ( b ) CR-enhanced embedded state. During imaging, paraformaldehyde-fixed brain slices were kept in phosphate-buffered saline (0.01 M, pH=7.4); the corresponding LR White-embedded brain slices were kept in Na 2 CO 3 solution (0.1 M, pH=11.6). All images were acquired on the same microscope (Nikon A1) with the same configuration at 25 ° C (room temperature). Image dimensions of b were enlarged 1.34-fold to correct for the shrinkage caused by the embedding procedure. Intermediate dendrites are abbreviated (grey bands with dashed lines) to allow a much closer view of the details. Images of one apical dendrite were recorded before ( c ) and after ( d ) embedding to allow direct comparison of dendritic spine morphology. ( e , f ) Enlargements of insets (white boxes) from a , b . I 0 and I represent the integration of fluorescence intensities in the corresponding white circle. Fluorescence intensities of pixels crossed by the red and blue lines are plotted ( g ) as curves of the corresponding colour. ( h ) The EYFP preservation ratio. At least 15 mushroom spines were measured for every subregion. Error bars represent s.d.’s. ( i ) Statistics of dendritic spines and collateral boutons before and after embedding. Spines were counted on a portion of apical dendrites (ADs); boutons were counted in a 100 × 100 × 75 μm 3 layer (measured in the fixed state) containing axon collaterals (AC)s concentrated at three depth intervals (0–20, 20–40 and 40–75 μm). Deep-coloured pillars represent the PFA-fixed state, and light-coloured pillars represent the CR-enhanced resin-embedded state. Error bars represent the number of boutons with uncertain identification. All images are shown with the same colour bar except for c , d . Scale bar: ( a , b ) 40 μm; ( c , d ) 10 μm; ( e , f ) 2 μm. Full size image It should be noted that not only the Na 2 CO 3 buffer but also many alkalis also induced CR effect. We have first observed the same fluorescence recovery effect induced by NaOH solution, and then by those amines, such as NH 3 solution, NH 2 CH 2 CH 2 NH 2 solution, and even by those cationic surfactants, such as Cetyltrimethylammonium hydroxide. All these alkaline solutions (at a pH range from 9 to 12) present the same fluorescence recovery ability. Evaluation of structure preservation The uniformly high preservation ratios of EYFP and EGFP enable reliable detection of labelled structures in resin-embedded tissue. A group of integral layer V pyramidal neurons was visualized under high saturation conditions to reveal most of the detectable labelled structures. A sophisticated comparison along the whole neuron extension shows no discernable loss of detail ( Fig. 2a,b ). Meticulous comparison of the fine structures shows that the amount of signal and the morphological detail were both perfectly preserved; dendritic spines and collateral bouton counts in surface structures (within a 20-μm surface layer) show no notable differences between the resin-embedded state and the control state ( Fig. 2i ). CR does not create any obvious morphological differences in dendritic spines ( Fig. 2c,d ). By imaging and quantitatively comparing the same structures before and after resin embedding, we have demonstrated that the originally labelled structure can be faithfully visualized when embedded in resin. We observed that many more structures were detected in the CR-enhanced resin-embedded state. This is because the resin embedding causes several physical changes in the labelled tissues, which enable better fluorescence detection. First, the resin-embedding procedure can increase fluorescence because of tissue shrinkage. For MMA-embedded tissue, we observed 1.3- to 1.4-fold shrinkage uniformly in every dimension ( Fig. 3a,b ). This shrinkage causes the fluorophore density to increase. The high refractive index of resin-embedded tissue also increases the numerical aperture. In addition, the CR procedure results in ~0.28-fold more chromophores in the fluorescent state than in the original PFA-fixed tissue. As a result, the fluorescence intensity increases to 2.5 times its original value after PFA fixation ( Fig. 2e–g ). The resin-embedding procedure also improves the refractive index uniformity, which decreases the scattering interference. The tissue was partially transparent ( Supplementary Fig. 7a–d ). We have measured the transmittances of the brain slices at different states. At the original PFA-fixed state, the transmittance of a 100-μm-thick brain slice is only 20% at 488 nm; however, when it has been resin-embedded and CR-enhanced, it allows 83% transmittance of the 488-nm excitation light ( Supplementary Fig. 7f ). This makes it possible to see much deeper compared with the original fixed state. We counted axon collateral boutons in a surface layer region with a volume of 100 × 100 × 75 μm 3 (measured in the fixed state). The number of boutons detected in the fixed state decreased sharply and the identification uncertainty increased as imaging depth increased; however, this phenomenon does not noticeably occur in the embedded state ( Fig. 3i ). CR-enhanced ex vivo mouse brain imaging We further demonstrate that CR-enhanced resin-embedded fluorescence imaging can be used to study fluorescently labelled large tissue blocks and even whole mouse brains because of the good sectioning properties of resin embedding and CR-induced fluorescence recovery. A transgenic mouse, thy1-YFPH, was used as a model (see Supplementary Method for the whole-brain-embedding protocol). A subset of the projection neurons expressing thy1 in this mouse are labelled by EYFP [28] . The neural circuit paths across different brain areas are reconstructed accurately in three-dimensions (3D) at single-fibre resolution ( Fig. 4a and Supplementary Video 1 ). 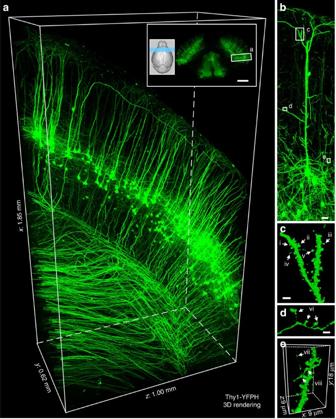Figure 4: Imaging of the thy1-YFPH mouse brain. (a) 3D presentation of a P21 thy1-YFPH mouse brain data set. Images were acquired with a voxel size of 0.5 × 0.5 × 1 μm3. The inset image shows the contours of the whole mouse brain, reconstructed by autofluorescence and coronal plane sectioning on the blue labelled region (centred at the bregma +1.50 level). Structures of the cerebral cortex are highlighted (white boxing inset) and enlarged to show details. Thezaxis represents the buffer penetration direction. (b) A layer V pyramidal neuron recorded at a 0.2 × 0.2 × 0.2 μm3voxel size on a commercial confocal microscope (Zeiss, LSM710).c–eshow enlargements of the fine structures from the white box region ofb. White arrows and numerals indicate (i) stubby, (ii) branched, (iii) thin, (iv) filopodium and (v) mushroom spines, as well as (vi)terminauxboutons, (vii)en passantbouton and (viii) structures suspected as synaptic connections. Scale bar: (a) inset, 1 mm; (b), 20 μm; (c,d), 2 μm. Dimensions: (a) 1,850 × 620 × 1,000 μm3; (e) 9 × 18 × 9 μm3. Figure 4: Imaging of the thy1-YFPH mouse brain. ( a ) 3D presentation of a P21 thy1-YFPH mouse brain data set. Images were acquired with a voxel size of 0.5 × 0.5 × 1 μm 3 . The inset image shows the contours of the whole mouse brain, reconstructed by autofluorescence and coronal plane sectioning on the blue labelled region (centred at the bregma +1.50 level). Structures of the cerebral cortex are highlighted (white boxing inset) and enlarged to show details. The z axis represents the buffer penetration direction. ( b ) A layer V pyramidal neuron recorded at a 0.2 × 0.2 × 0.2 μm 3 voxel size on a commercial confocal microscope (Zeiss, LSM710). c – e show enlargements of the fine structures from the white box region of b . White arrows and numerals indicate (i) stubby, (ii) branched, (iii) thin, (iv) filopodium and (v) mushroom spines, as well as (vi) terminaux boutons, (vii) en passant bouton and (viii) structures suspected as synaptic connections. Scale bar: ( a ) inset, 1 mm; ( b ), 20 μm; ( c , d ), 2 μm. Dimensions: ( a ) 1,850 × 620 × 1,000 μm 3 ; ( e ) 9 × 18 × 9 μm 3 . Full size image The two-photon fluorescence micro-optical sectioning tomography (2 P-fMOST) system [29] , which combines a microtome and the two-photon microscope to enable successive block-face imaging, has been used to implement this task. To induce sufficient CR during the imaging procedure, a water immersion objective was used, and alkaline buffer was used as the immersion medium, which made it possible to continue penetrating the specimen’s block-face during imaging. Successive measurements of the penetration rate show that the relationship between penetration time and reactivating layer thickness is a quadratic function, which obeys the diffusion equation for a liquid diffusing in a semi-infinite homogeneous solid [30] ( Supplementary Discussion 1 and Supplementary Fig. 8 ). This diffusion law enables us to reliably estimate the penetration thickness for a given imaging time. By matching the periodical resection thickness with the imaging speed, we successfully ensured that the layers photographed were within the portion of tissue that was sufficiently penetrated by the buffer, thus ensuring uniform fluorescence intensity along the depth direction. A whole-brain data set with 0.5 × 0.5 × 1 μm 3 voxel size was acquired after 2 weeks of successive imaging by this strategy. The 3D reconstruction results illustrate that throughout the ~40-mm 2 scope focal planes, and within several millimetres in the depth direction, the fluorescence intensities of the structures are quite uniform ( Fig. 4a and Supplementary Discussion 2 ). To enable a much more intuitive experience of the fine structure on a much larger scale, we created a movie that simulates travelling through the brain from the cortex to the corpus callosum by following the axon stream ( Supplementary Video 1 ). Actually, the 0.5 × 0.5 × 1 μm 3 sample rate of the whole-brain data set is not sufficient to display some important structural details that may be of interest to many neuroanatomists, such as the dendritic spines and axon terminals. To fully reveal these fine structures, we have performed imaging with another CR-enhanced specimen (an LR White-embedded thick section) using a much higher sample rate (0.2 × 0.2 × 0.2 μm 3 ) on a commercial confocal microscope (Zeiss, LSM710; Fig. 4b–e ). Along the extension of a layer V pyramidal neuron, we observed all five types of dendritic spines with ultrahigh contrast: thin, stubby, mushroom, filopodium and branched spines ( Fig. 4b,c ) [27] , [31] . The presynaptic structures, terminaux boutons and en passant boutons [32] , [33] can be clearly identified along the axon collaterals, distributed across the field of view ( Fig. 4b,d ). Structures suspected as synaptic connections can also be frequently detected along the dendrites ( Fig. 4b,e ). The CR phenomenon described here allows the resin-embedding method to be compatible with powerful fluorescent-labelling techniques based on GFP. We found that using the normal embedding procedure, most GFP molecules are preserved in a nonfluorescent state by chromophore protonation, rather than directly damaged, and can be chemically recovered to their fluorescent state by our CR method during imaging. The effect of CR is not dependent on expression host. Our findings thus enable imaging of resin-embedded fluorescent protein-labelled tissues without noticeable loss of labelled structures. It is well known that the unusually stable β-barrel structure of GFP and its derivatives protect against denaturation, proteolysis and chromophore oxidation/reduction by exogenous molecules [6] , [34] . Actually, most of the commonly used fluorescent proteins [35] , either derived from AGFP or derived from DsRed, share the same β-barrel overall fold [34] , [36] . Perhaps the most significant discovery we describe here is that this basic β-barrel structure survives the acryl resin-embedding procedure and maintains its functionality. Our absorption spectrum study shows that GFP denaturation is not significant, and the high fluorescent protein preservation ratios indicate that the chromophores are well protected from the radical polymerization reactions by the wonderful β-barrel. This discovery indicates that these commonly used fluorescent proteins can be structurally preserved in acryl resins. Fluorescent proteins with protonation-sensitive chromophores have to be reactivated by our CR method, such as those GFP and yellow–green-fluorescent proteins (EGFP, EYFP, mCitrine, Venus and YPet and so on) derived from AGFP, and orange-fluorescent proteins (mOrange, mKO and so on) derived from DsRed. Fluorescent proteins with protonation-insensitive chromophores can be directly preserved in those acryl resins, such as those famous red-fluorescent proteins (mCherry, mStrawberry and so on) derived from DsRed. We have verified that mCherry can be well preserved in GMA- and MMA-embedded mouse brains ( Supplementary Fig. 9 ). In addition, CR processing has no effect on it. These results on EYFP, EGFP and mCherry directly support this prediction. In previous researches for retaining fluorescence in resin-embedded samples, methods based on ultra-low-temperature freezing, freeze substitution and polymerization have enabled successful detection and analysis of GFP fluorescence in cultured cells and small tissues [7] , [8] , [9] . However, besides still experiencing quenching, these methods can hardly transplant for macroscopic tissue block embedding. As the freezing and freeze substitution techniques applied cannot process tissue blocks thicker than 0.6 mm [37] , [38] and, in the meantime, the UV light used for low-temperature polymerization has limited penetration depth. LR White-embedded small plant tissues has been reported to retain 72.5% GFP fluorescence [10] ; however, similar experiments on animal tissues do not acquire such high fluorescence preservation [11] , [12] , [13] . Without the guidance of an identified mechanism that describes the behaviours of fluorescent protein molecules during resin embedding, previous efforts on macroscopic tissue embedding have focused on empirically optimizing the resin-embedding procedure before polymerization, for example, by optimizing the dehydration degree of the tissue [12] , the water content or the pH of the embedding medium [13] . However, only limited success can be achieved in optimizations of these pre-polymerization processes. These previous optimization methods necessitate a compromise between providing ideal polymerization conditions and maintaining GFP fluorescence. Embedding protocols cannot always be suitably modified to enable preservation of most of the fluorescent protein molecules. For instance, mixing the embedding medium with water or alkaline solution is thought to improve fluorescence intensity [8] , [13] ; however, to maintain effective polymerization, the amount of water or buffer added must not exceed 5%, which is insufficient to achieve good fluorescence preservation [8] . Furthermore, empirical methods are always difficult to transplant for preservation of other fluorescent proteins. As a specimen preparation method for microscopic imaging, resin embedding facilitates good cutting performance. It enables microimaging with homogenous high resolution across a whole organ or animal by successive removal of layers, without alignment problems because of distortion [39] . The single-fibre continuity that can be observed in the whole thy1-YFPH mouse brain data set benefits greatly from this technique. It is noted that the very surface layer (several micron level) of the resin-embedded tissue block indeed has changed when soaked into water, although the bulk hardness keeps stable ( Supplementary Table 1 ). It swells slightly when compared with the dry state. However, the swelling does not affect the successive semi-thin sectioning with thickness ranges from 500 nm to 2 μm in 2 P-fMOST imaging. When ultrathin sections are needed, CR can be used during imaging, after the slices have been collected. CR buffer penetration also influences the optical property of penetrated portion of the resin-embedded tissues. For example, sufficient buffer penetration introduces a little bit of transparency deterioration ( Supplementary Fig. 7e ). However, this kind of optical property change does not affect thick tissue imaging described here, with the help of successive semi-thin sectioning and block-face imaging. It is also noted that in the demonstration we chose a P21 thy1-YFPH mouse brain to show a moderate neuronal fibre density distinguishable under optical microscopy. We tried it in older mice (P45) and observed similar fluorescence enhancement with CR; however, the brain has very high density of neurons expressing EYFP—fibres (especially the axon collateral) entangled together cannot be distinguished with normal optical microscopy ( Supplementary Fig. 10 ). Resin embedding and fluorescent protein labelling are both widely used techniques in biology and medicine; therefore, we believe that the method presented here provides a valuable bridge between two important methods that were previously incompatible. This may enable new types of studies and breakthroughs in the future. For example, CR may provide a convenient way to combine fluorescence microscopy and electron microscopy at a much macroscopic scale. If it becomes easy to match interesting protein expression patterns to the corresponding local cellular ultrastructure components with great spatial range, a new level of understanding will be possible for cell biologists. Animal selection We chose the most widely used GFP tag and GFP variants to use as fluorescence markers for validation. Approximately 20 female thy1-YFP-H P21 mice (JAX stock number 003782) and 15 female thy1-EGFP-M P60 mice [28] (JAX stock number 007788) were used in this study. One thy1-YFP-H P21 female mouse and another thy1-EGFP-M P60 female mouse was used for fluorescent protein preservation evaluation and pKa measurement: the animals were first fixed by transcardial perfusion and sliced to 75 μ coronal plane slices by a vibration microtome (Leica, VT1000 S); slices that have relatively integral Layer V pyramidal neurons were used for confocal imaging before and after resin embedding. To demonstrate that our CR-enhanced specimen provide good stability and uniform fluorescence intensity for long time microscopic specimen imaging, one thy1-YFP-H P21 female mouse was used for whole-brain serial block-face two-photon imaging. The remaining mice were used for protocol test and CR effect evaluation on different embedding media. All procedures were approved by the Institutional Animal Ethics Committee of the Huazhong University of Science and Technology. pKa measurement The pKa of EYFP in PFA-fixed tissue has been measured. Several pieces of 75 μ-thick coronal plane slices of PFA-fixed thy1-YFPH mouse brain have been used. First, we modified the pH of 0.01 M PBS (pH=7.40, pH measured by a pH meter, accurate to two decimal places) by NaOH to prepare PBS buffers with different pH (from 7.40 to 10.40, 0.50 increase per step). Imaging brain slices in these buffers show that when pH reached 9.40, the fluorescence intensity of the fixed tissue reached the maximum. In addition, it shows little difference with the intensity imaged in buffer of pH=8.90. Fluorescence intensity ratios of 94 mushroom spines between pH=7.40 and pH=9.40 have been measured. Fluorescence intensity was regarded as the intensity integration over whole spine bodies. Their distribution was fitted to a normal distribution. We used the mean value estimates of the distribution as the measured fluorescence intensity ratio, denoted as R , and then the pKa can be represented as . Specimen preparation Several thy1-YFP-H P21 and thy1-EGFP-M P60 mouse brains were embedded with LR White (Structure Probe Inc.), GMA (Technovit 8100, Electron Microscopy Sciences) or MMA (Technovit 9100, Electron Microscopy Sciences). The transcardially perfused mouse brains were first removed from the skull and transferred to neutral buffered PFA (4% w/v in 0.01 M PBS, 50 ml per brain) for ~12 h post fixation. After post fixation, we moved the mouse brain to fresh 0.01 MPBS for a 12 h rinse (50 ml per mouse brain). For LR White- and GMA-embedded specimens, a graded series of ethanol solutions was used to dehydrate the tissue (four solutions were used: 50, 75, 95% and a second 95% treatment (w/w), each incubated for 1 h). The mouse brain exhibited slight shrinkage. After dehydration, the samples were ready for infiltration: they were successively soaked in a graded series of infiltration solutions (50, 75, 100 and 100% embedding medium in 95% ethanol, 2 h each for the first three solutions and 48 h for the final solution). The specimens were transferred to gelatin capsules and immersed in LR White or GMA polymerization solution. The LR White capsules were cured at 55 ° C for 5–7 h. The GMA capsules were transferred to a 4 ° C refrigerator for ~12 h of polymerization. For MMA embedding, the mouse brain must be completely dehydrated; therefore, the ethanol gradient and incubation times were adjusted as follows: five incubations with 50, 75, 95, 100% and 100% ethanol, 2 h each. After dehydration, the dehydrated brain was immediately cleared twice in xylene (50 ml per brain) for ~2 h each time. The brain should be rendered totally transparent by the xylene. After this, the specimen can be infiltrated by infiltration solutions and stock solution A, which is described by the data sheet (all solutions were prepared using destabilized basic solution, and the last infiltration was performed for at least 48 h). We used a version of stock solution A that is slightly different from what the data sheet advised: we used only half of the suggested amount of PMMA (polymethyl methacrylate) powder to ensure optimal preservation of structural morphology in the soft tissue. For polymerization, specimens were transferred into gelatin capsules and immersed in polymerization solution; however, as MMA (Technovit 9100) embedding medium is anaerobic before polymerization, the capsule should be opened and kept under vacuum at 4 ° C for ~10 min. Only after this procedure can the capsules be closed and moved into a −4 ° C dark and dry chamber for 72 h of polymerization. All soaking and infiltration steps for these specimens were conducted at 4 ° C in the dark. We used experiments on mouse brain slices to determine how well CR preserves the structure and fluorescence of soft tissue sections. To ensure that our experiments on brain slices can be generalized to whole mouse brains, we used the same protocol for 75 μ brain slice embedding as for whole-mouse brain preparation, as stated above. Absorption spectrum measurement The recombinant EGFP we used was the histidine-tagged fusion protein of GFP that was expressed in E. coli and purified by nickel-chelate affinity chromatography [21] , [40] . All the absorption spectra were measured on the LAMBDA 950 UV/Vis/NIR Spectrophotometer (PerkinElmer), with a 1-nm spectral resolution. Absorption spectra of recombination EGFP in solutions (0.01 M PBS buffer, pH=7.4 and PBS buffer titrated by HAC, pH=5.0) has been measured as the controls. Then recombination EGFP solution has been dialysed in distilled water to remove the salts. Since EGFP cannot efficiently dissolve in resin monomer, resin sheet that polymerized on glass slides had been prepared, and the EGFP protein solution was spread and dried (in vacuum) on these sheets. When absorption spectrum of EGFP in resin monomer was measured, 100 μl resin monomer was added on this EGFP-absorbed resin sheet, and a coverslip was covered on it immediately to prevent monomer evaporation and, after 30-min incubation, the spectrum was measured. When absorption spectrum of EGFP embedded in resin was measured, 40 μl embedding solution was added on this EGFP-absorbed resin sheet, and a coverslip was covered immediately to exclude the air. The spectrum can be measured after polymerization. It should be noted that LR White must be polymerized in vacuum at 55 ° C to enable sufficient polymerization. When absorption spectrum of EGFP after fluorescence recovery was measured, the coverslip of the polymerized sheet was removed, and the sheet was soaked in 0.001 M NaOH for at least 4 days under dark condition. The spectrum should be measured after sufficient penetration. All the absorption spectra were normalized at the 429 nm osbestic point measured at solution condition for further analysis. Fluorescence spectrum measurement All the fluorescence spectra were directly measured on the thy1-YFPH or thy1-GFPM mouse brain tissues (resin-embedded or PFA-fixed) by the commercial confocal microscope (Zeiss, LSM710), with a 3.4-nm spectral resolution. The EYFP was excited by 514 nm laser, and the EGFP was excited by 488 nm laser. Confocal imaging To reveal the CR phenomenon on the solid–liquid surface, entire LR white-, GMA- and MMA- embedded mouse brains were used. The brains were first trimmed to reveal the coronal plane (approximate bregma +1 level) by a diamond knife (ultra 45 ° , Diatome) at dry state. Before imaging, the diamond-machined surface was penetrated by alkaline buffer (0.1 M Na 2 CO 3 solution, pH=11.6) for 2 min; then the surface was immediately immersed into oil and imaged with a 60 × 1.4 NA oil immersion objective (CFI Plan Apo, Nikon). We used a commercial confocal microscope (A1, Nikon) to implement this imaging task. For every specimen, axon bunches that extend downwards at the striatum region were imaged to enable a convenient quantification of the CR-induced fluorescence enhancement. Microscope was configured to scan stepping into the diamond-machined surface 0.2 μm per slice to acquire a 60 μm z-stack. To evaluation the CR-enhanced resin-embedded fluorescent protein-labelled tissue, the 75 μ-thick brain slices were immediately imaged by an inverted commercial confocal microscope (A1, Nikon) once it has been prepared. The slices that have not been embedded were first imaged in sample cell that was filled with PBS (0.01 M, pH=7.4, Sigma) at 25 ° C temperature. In addition, the 60 × 1.4 NA oil immersion objective (CFI Plan Apo, Nikon) is used to ensure good distinguishability of the dendritic spines and collateral buttons. To ensure a maximum revealing of the fine structure, the microscope was configured with 6% laser power (Exited by 488 nm wavelength laser), 0.21 × 0.21 μm 2 pixel size, 110 V PMT voltage and 2,400 ns pixel dwell time. Several relatively integral Layer V pyramidal neurons were imaged by this configuration; the imaging followed the neurons’ extension from the apical dendrite region to the ventral pallidum. Then the imaged brain slices were embedded between two coverslips, before being reimaged, and the embedded brain slices were removed from the coverslips by soaking it in our penetration buffer (0.1 M Na 2 CO 3 solution, pH=11.6). The brain slices can be easily removed when they were sufficiently penetrated. These sufficiently penetrated embedded brain slices were then moved into the same sample cell that filled with penetration buffer for reimaging. The microscope was set to the same configuration as the slices were first imaged. Successive two-photon block-face imaging A LR White-embedded P21 thy1-YFPH mouse brain was imaged. The successive imaging procedure was implemented as follows: first, a water immersion objective was used and alkaline buffer was used as the immersion medium. The resin-embedded mouse brain was fixed and soaked in the immersion medium and a fine plane was previously machine-cut in parallel with the focal plan using a diamond knife. Scanning microscopy with a 3D moving stage was used to record images for the desired thickness representing the activated layer of the specimen surface. After each image was recorded, the moving stage drove the specimen towards a fixed diamond knife to remove the recorded layer. This process was repeated for each imaging cycle. The buffer solution was allowed to penetrate during each imaging cycle, and the removal of the layer thickness matched the imaging speeds that, at the start of each image cycle, the buffer had already penetrated through to the appropriate thickness. Imaging cycles were repeated until the entire specimen was processed. The moving stage remembers the coordinates of the acquired images and uses them for 3D reconstruction. We used 2 P-fMOST [29] to implement this strategy. Before imaging, one end of the resin-embedded specimen cylinder was flattened and stuck to our custom-made copper specimen holder. The glue was allowed to dry (cyanoacrylate glue, Fisher Scientific) and the specimen was milled to the olfactory bulb position for diamond knife trimming. After trimming, the finely machined plane was used for CR. The specimen was transferred into a plastic container and fixed on the holder with four screws. A solution of 0.1 M Na 2 CO 3 (pH=11.6) was transfused into the container to serve as an immersion medium for the water immersion objective (UPLAN 40 × 0.75 NA, Olympus). This alkaline immersion medium immediately penetrated into the finely machined plane and activated a micron-scale enhanced fluorescence layer. The penetration time is a quadratic function of the penetration thickness, and we found that the hydrophilic nature of the embedding medium also affects penetration. For the hydrophilic embedding media that we tested (LR White and GMA), 1 min of penetration results in an enhanced fluorescence layer ~5-μ thick, but the penetrated layer was only ~2-μ thick when the hydrophobic Technovit 9100 medium was used. For successive block-face imaging, we set the focus of the two-photon microscope to 3 μ below the diamond knife-machined surface, and each imaging cycle contained six coronal plane layers (1 μm per layer). The penetration speed is fast enough for successive imaging: the fastest our imaging system can go is 300 ns per pixel; for a 0.5 μm × 0.5 μm pixel size and a 1 μm axial step size, it takes 2–4 min to acquire a whole coronal plane for a single step (the coronal plane dimensions change gradually, so the imaging times varies). The alkaline immersion medium penetrates ~10 μ in the LR White-embedded mouse brain. Thus, it consistently showed uniform fluorescence enhancement during the 2-week data acquisition period. A 50-mW laser (925 nm wavelength, 140 fs pulse width) beneath the objective was used to ensure high contrast for the main axons of the projection neurons. Quantification of CR Main axons that penetrated the 60-μm z-stack were randomly selected to evaluate CR-induced fluorescence intensity enhancement in tissue blocks embedded by different embedding media. The maximum fluorescence intensity of each axon in each layer was identified using the measurement tool in ImageJ. For each data set from the different resin-embedded tissue blocks, we averaged the intensities of axons to remove intensity fluctuations caused by structural differences and axon extension orientation differences. This normalized average intensity was fitted to the normalized solution of diffusion equation by the least-squares fitting method. The normalized solution of diffusion equation can be written as, Here n represents the Nature Numbers, which are corresponding to the image no. in the z-stack (1 represents the layer no. with the highest fluorescence intensity, the no. increases as the image goes deep into the penetration surface). C 1 represents the initial fluorescence intensity before penetration. C 2 is a constant decided by diffusion coefficient and the penetration time. The reciprocal of C 1 represents the CR-induced fluorescence enhancement factor. Preservation analysis Data sets of brain slice images were used for the preservation study of tissue structure and protein fluorescence. To evaluate the preservation of fluorescence, mushroom spines unsaturated before and after resin embedding were selected and used for fluorescence intensity comparisons. The grey values of all pixels in a mushroom spine head were summed to represent the total fluorescent intensity of the spine [8] , which is denoted as I 0 for the PFA-fixed state and I for the CR-enhanced resin-embedded state. For the fixed state EYFP-labelled tissue, the total number of EYFP molecules in a mushroom spine is 1.28 I 0 . For fixed state EGFP-labelled tissue, the total number of EGFP molecules in a mushroom spine is just I 0 . Thus, the fluorescent protein preservation ratio of a mushroom spine is I /(1.28 I 0 ) for EYFP-labelled tissue and I / I 0 for EGFP-labelled tissue. We used 87 mushroom spines to determine the preservation ratios in LR White-embedded EYFP-labelled tissue. The distribution of preservation ratios was fitted to a normal distribution, and the mean value of the distribution was taken to be the fluorescent protein preservation ratio. To evaluate structure preservation, we counted dendritic spines on a portion of an apical dendrite that had images representing both states, and we checked to see whether the spines were preserved in the CR-enhanced specimens. Axon boutons were also counted in a 100 × 100 × 75 μm layer containing concentrated axon collaterals. The boutons and spines that could not be identified by either of two professional researchers were considered to be ‘uncertain.’ Image 3D reconstruction 3D reconstructions were implemented by transforming the image stack into Large Data Access using the Amira software (Visage Software, San Diego, CA, USA). Further analysis guidance can be found in other published methods [41] . How to cite this article : Xiong, H. et al. Chemical reactivation of quenched fluorescent protein molecules enables resin-embedded fluorescence microimaging. Nat. Commun. 5:3992 doi: 10.1038/ncomms4992 (2014).